Arthropod fossil data increase congruence of morphological and molecular phylogenies The relationships of major arthropod clades have long been contentious, but refinements in molecular phylogenetics underpin an emerging consensus. Nevertheless, molecular phylogenies have recovered topologies that morphological phylogenies have not, including the placement of hexapods within a paraphyletic Crustacea, and an alliance between myriapods and chelicerates. Here we show enhanced congruence between molecular and morphological phylogenies based on 753 morphological characters for 309 fossil and Recent panarthropods. We resolve hexapods within Crustacea, with remipedes as their closest extant relatives, and show that the traditionally close relationship between myriapods and hexapods is an artefact of convergent character acquisition during terrestrialisation. The inclusion of fossil morphology mitigates long-branch artefacts as exemplified by pycnogonids: when fossils are included, they resolve with euchelicerates rather than as a sister taxon to all other euarthropods. Arthropods are diverse, disparate, abundant and ubiquitous; they outnumber all other animal phyla combined. Five major extant groups can be distinguished ( Fig. 1 ): pycnogonids (sea spiders), euchelicerates (horseshoe crabs and arachnids), myriapods (centipedes and millipedes), hexapods (insects and their flightless relatives) and crustaceans (crabs, lobsters, barnacles and so on). Each group is characterized by a distinct set of morphological features and their monophyly is little disputed, except for the crustaceans [1] , [2] , [3] , [4] . Molecular clock estimates calibrated by new fossil discoveries indicate that these groups originated and had begun to diversify by at least the mid-Cambrian [5] . Hence, they have had more than 500 million years to specialize and overprint ancestral characteristics, and thus few unequivocal features are informative with regards to their interrelationships. Molecular characters provide an alternative source of data that has partly alleviated this problem, although some resultant trees have recovered groupings with little morphological support. An example is a clade comprising chelicerates (pycnogonids and euchelicerates) and myriapods as sister taxa [6] , [7] , [8] , [9] ( Fig. 1a ), considered so surprising it was named Paradoxopoda [8] (alternatively Myriochelata [9] ). Although a few neuroanatomical and developmental characters were later proposed as putative novelties of Paradoxopoda [10] , [11] , subsequent exploration of molecular data sets suggested that this grouping is a long-branch artefact [3] , [12] . 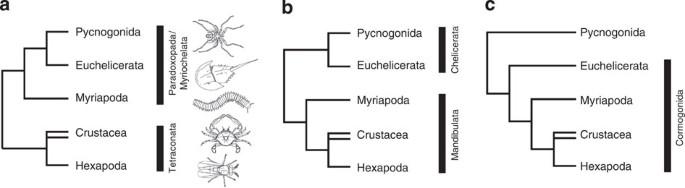Figure 1: Current hypotheses of arthropod interrelationships. (a) Paradoxopoda (Myriochelata) hypothesis with myriapods as sister taxon to Chelicerata. (b) Chelicerata/Mandibulata hypothesis with a clade composed of euchelicerates and pycnogonids (Chelicerata) as sister taxon to Mandibulata. (c) Cormogonida hypothesis with pycnogonids as sister taxon to all other euarthropods (Cormogonida). Figure 1: Current hypotheses of arthropod interrelationships. ( a ) Paradoxopoda (Myriochelata) hypothesis with myriapods as sister taxon to Chelicerata. ( b ) Chelicerata/Mandibulata hypothesis with a clade composed of euchelicerates and pycnogonids (Chelicerata) as sister taxon to Mandibulata. ( c ) Cormogonida hypothesis with pycnogonids as sister taxon to all other euarthropods (Cormogonida). Full size image Diverse molecular data sources support a close relationship between hexapods and crustaceans (collectively known as Tetraconata or Pancrustacea), either as sister taxa [6] , a result also favoured by some morphological evidence [13] , [14] , or more typically with hexapods nested within a paraphyletic Crustacea. The latter is supported by a number of independent lines of evidence, including nuclear ribosomal genes [8] , [15] , mitochondrial genomes and gene order, nuclear protein-coding genes [1] and transcriptomics [2] , [3] , [4] , but has so far remained elusive in morphological phylogenies, apart from those based solely on neural characters [16] , which resolve malacostracan crustaceans closer to hexapods than to branchiopods. The position of the pycnogonids is equally controversial, being variously resolved as the closest relatives of euchelicerates [1] , [3] , [15] ( Fig. 1a,b ) or as sister taxon to all other euarthropods [17] ( Fig. 1c ; the ‘Cormogonida hypothesis’). The relative paucity of Recent morphological characters that unite pycnogonids with other arthropods or unite hexapods with any particular crustacean group to the exclusion of other groups has hampered attempts to remove long-branch artefacts and decide between alternative hypotheses. Inclusion of fossil taxa, however, provides a possible mechanism for sampling ancestral morphologies and extinct character combinations; fossil morphology has been shown in other phylogenies to mitigate long-branch biases [18] , [19] . For this reason, we undertook a large-scale phylogenetic analysis that incorporates data from a total of 309 panarthropods (plus two non-panarthropod ecdysozoans), including all major extinct and extant panarthropod groups. The 753 characters primarily describe morphology (703 characters), but are supplemented with additional data from development (29 characters), behaviour (6 characters) and gene order and gene expression (15 characters). The latter were included because they are analysed like morphology (amenable to absence/presence coding) rather than like sequence data. These characters were optimized using both equal character weighting and implied character weighting [20] with a range of concavity constants ( k =2, 3 and 10). Compared with previous morphology-based analyses [24] , this study more than doubles the number of fossil terminals ( n =215). For the first time, the sample of fossil taxa includes most of the best-known arthropods from all major Cambrian to Devonian Konservat Lagerstätten, including Chengjiang, Sirius Passet, the Emu Bay Shale, the Burgess Shale, Swedish Orsten, Herefordshire and Hunsrück. This analysis demonstrates the importance of including fossil data in large-scale phylogenetic analyses and helps to resolve long-standing conflicts regarding the relationships of crown-group arthropods. The plesiomorphic condition of Euarthropoda Each analysis recovered a fundamental split in the arthropod crown group (Euarthropoda) between Chelicerata and Mandibulata (myriapods, hexapods and crustaceans); both of these two main clades have a diverse fossil stem group ( Fig. 2 ). The mandibulate stem group is composed of marrellomorphs, Agnostus , and a variety of other Cambrian Orsten taxa, including phosphatocopines. Successive outgroups of Chelicerata include vicissicaudates (aglaspidids, cheloniellids, xenopods and Sanctacaris ) and a paraphyletic assemblage of trilobitomorphs. Most of these taxa (including trilobites) have traditionally been regarded as stem chelicerates under the Arachnomorpha hypothesis [21] , [22] , but more recent hypotheses regarding the organization of the arthropod head prompted their assignment to total-group Mandibulata [23] . These and some subsequent studies considered deutocerebral antennae to be an autapomorphy of total-group Mandibulata and the raptorial first pair of appendages of pycnogonids and euchelicerates to be a symplesiomorphy of Euarthropoda [19] , [24] . Under this scheme, the raptorial appendages of stem-group euarthropods such as megacheirans (‘great-appendage’ arthropods), fuxianhuiiids and bivalved stem-group arthropods (for example, Odaraia , Canadaspis and Perspicaris ) were considered homologous to the chelicerae of chelicerates, and any antenniform appendages anterior to this were considered segmentally homologous to the antennae of onychophorans, that is, protocerebral rather than deutocerebral. Recent studies of Fuxianhuia and other closely related taxa [25] , [26] , however, indicate that the antennae are in fact deutocerebral. This finding implies that their post-antennal appendages are not homologous to chelicerae, and that mandibulate antennae are homologous to the antennae of many or most members of the euarthropod stem group. Our analyses resolve deutocerebral antennae as the symplesiomorphic condition for Euarthropoda, with chelicerae being a transformation of them and an unequivocal autapomorphy of Chelicerata ( Fig. 2 ). 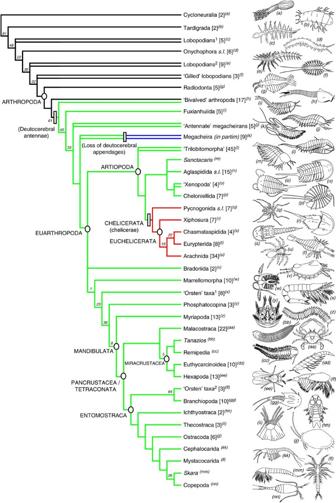Figure 2: Summary of relationships amongst major arthropod taxa based on 311 taxa and 753 characters. A summary of all results produced using implied weighting (k=2, 3 and 10). The equally weighted tree differs mainly in the position of hexapods, which resolve as sister taxon to all other pancrustaceans (monophyletic Crustacea). A full tree showing the position of all terminals is presented inFig. 4. Paraphyletic taxa are indicated with a double line, numbers in parentheses indicate the number of terminals analysed within each group. Colours on branches show the transformation between antennae and chelicerae. Lineages possessing an anterior (presumably deutocerebral) pair of antennae are indicated in green, chelierate-bearing lineages in red, taxa which have secondarily lost their deutocerebral appendages in blue, and taxa lacking specialized arthropodized cephalic appendages in black. Numbers associated with nodes are selected Group present/Contradicted support values. Figure 2: Summary of relationships amongst major arthropod taxa based on 311 taxa and 753 characters. A summary of all results produced using implied weighting ( k =2, 3 and 10). The equally weighted tree differs mainly in the position of hexapods, which resolve as sister taxon to all other pancrustaceans (monophyletic Crustacea). A full tree showing the position of all terminals is presented in Fig. 4 . Paraphyletic taxa are indicated with a double line, numbers in parentheses indicate the number of terminals analysed within each group. Colours on branches show the transformation between antennae and chelicerae. Lineages possessing an anterior (presumably deutocerebral) pair of antennae are indicated in green, chelierate-bearing lineages in red, taxa which have secondarily lost their deutocerebral appendages in blue, and taxa lacking specialized arthropodized cephalic appendages in black. Numbers associated with nodes are selected Group present/Contradicted support values. Full size image The phylogenetic position of Pycnogonida Our phylogeny accordingly resolves pycnogonids and euchelicerates as sister taxa, although few characters beyond their shared chelicerae/chelifores support this placement. When fossils are removed from the data set (DS-II and DS-V; Table 1 ), pycnogonids are instead recovered as sister group of all other arthropods (Cormogonida) ( Fig. 3 ). Many characters supporting the monophyly of Cormogonida in this latter tree, such as the presence of a telson, occur in the pycnogonid stem lineage and, hence, do not support Cormogonida in the full analysis (DS-I). Our full analysis recovers a long stem lineage for the Euarthropoda ( Figs 2 and 4a,b ), comprising lobopodians, dinocaridids, bivalved arthropods, fuxianhuiids and megacheirans, consistent with a few previous analyses [24] , [27] . Many of the ‘typical’ euarthropod features, such as compound eyes, an arthrodized trunk, arthropodized limbs and specialised head appendages, were gradually acquired in the euarthropod stem lineage [24] ; when these stem-group exemplars were removed from the data set (DS-III), Cormogonida was again recovered ( Fig. 3 ). We hence interpret Cormogonida to result from an attraction between Euchelicerata and Mandibulata caused by the secondary reduction of typical euarthropod characters in pycnogonids. Table 1 Composition of data sets analysed in this study. 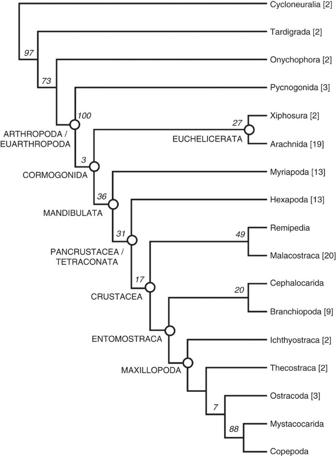Figure 3: Relationships amongst major arthropod taxa when fossils were removed from the data set. Numbers associated with nodes are Group present/Contradicted support values based on analyses using implied weighting (k=3). Numbers in parentheses indicate the number of taxa analysed within each group. Full size table Figure 3: Relationships amongst major arthropod taxa when fossils were removed from the data set. Numbers associated with nodes are Group present/Contradicted support values based on analyses using implied weighting ( k =3). Numbers in parentheses indicate the number of taxa analysed within each group. 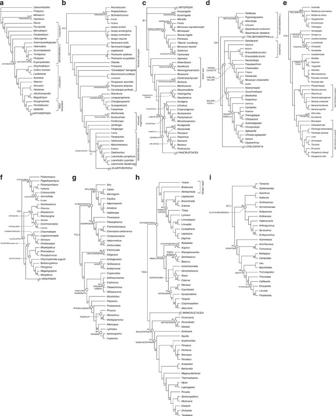Figure 4: Phylogeny of panarthropoda. Strict consensus of 45 MPTs (Most Parsimonious Trees) of 13,987,601 steps (adjusted homoplasy=592; consistency index (CI)=0.520, Retention index (RI)=0.873) produced using implied character weighting (k=3). Numbers associated with nodes are Group present/Contradicted support values. (a) Non-arthropod panarthropods and cycloneuralians. (b) Radiodontans and upper stem-group euarthropods. (c) Total-group Mandibulata and Bradoriida. (d) Stem-group chelicerates (Artiopoda). (e) Trilobitomorphasensu stricto. (f) Chelicerata (including Xiphosura and stem-group Arachnida). (g) Arachnida. (h) Pancrustacea. (i) Miracrustacea. Full size image Figure 4: Phylogeny of panarthropoda. Strict consensus of 45 MPTs (Most Parsimonious Trees) of 13,987,601 steps (adjusted homoplasy=592; consistency index (CI)=0.520, Retention index (RI)=0.873) produced using implied character weighting ( k =3). Numbers associated with nodes are Group present/Contradicted support values. ( a ) Non-arthropod panarthropods and cycloneuralians. ( b ) Radiodontans and upper stem-group euarthropods. ( c ) Total-group Mandibulata and Bradoriida. ( d ) Stem-group chelicerates (Artiopoda). ( e ) Trilobitomorpha sensu stricto . ( f ) Chelicerata (including Xiphosura and stem-group Arachnida). ( g ) Arachnida. ( h ) Pancrustacea. ( i ) Miracrustacea. Full size image The phylogenetic position of Hexapoda A sister-group relationship between Hexapoda and Crustacea is recovered in the extant-only ( Fig. 3 ) and equally weighted trees, but not in the full analysis with implied weights, where Crustacea is paraphyletic with respect to Hexapoda ( Figs 2 and 4h ). The latter result (crustacean paraphyly) arises from the use of methodologies that are more philosophically sound, that is, implied character weights rather than equal weights (see Methods for justification of implied weights), and more comprehensive taxon sampling, that is, including extinct and extant taxa rather than extant alone. When myriapods were removed from these data sets, the remipedes (plus the Silurian fossil Tanazios [28] in the total data set) resolved as the closest extant sister taxon to hexapods (and euthycarcinoids), thus retrieving crustacean paraphyly and mirroring the molecular support for a remipede sister group to hexapods [1] , [2] , [29] ( Fig. 3 ). Apomorphies for a clade of remipedes and hexapods (Miracrustacea in partim ) are in part influenced by character states in their fossil sister groups ( Tanzazios and euthycarcinoids), such as the apparent presence of an intercalary segment in Tanazios [30] versus a second antenna in extant remipedes, whereas others are sourced from internal anatomy of extant taxa [31] . Apomorphies of a remipede–hexapod clade are instead resolved as symplesiomorphic for Tetraconata in the extant-only data set (DS-II) because of their shared presence in myriapods. The total-evidence topology ( Figs 2 and 4 ) indicates that characters supporting a close relationship between myriapods and hexapods were convergently acquired. Among these are the presence of a limbless intercalary segment in the head, uniramous appendages, tracheae, Malpighian tubules as ectodermal extensions of the hindgut and a tentorial endoskeleton. Some of these are variously present in a number of other arthropods, such as uniramy of the cephalic appendages in extant arachnids. Some homoplasy may stem from common adaptation to a terrestrial environment; this was tested using selective deactivation of characters (DS-IV and DS-V; details in Methods). Those characters linked to a terrestrial ecology, such as uniramy, were found to have the greatest effect on topology (DS-IV) and their deactivation recovered topologies in which hexapods grouped with remipedes rather than with myriapods. We therefore conclude that crustacean monophyly is influenced by the convergent acquisition of terrestrial adaptations in myriapods and hexapods, with the result that crustaceans attract to each other when hexapods group with myriapods. The continued attraction between myriapods and hexapods in the equally weighted analyses may be due to the paucity of stem-group representatives of these lineages—although euthycarcinoids resolved as sister taxon to hexapods in the current study, they share few characters to place them unambiguously. These results are not biased by the inclusion of characters that have little or no fossilization potential, such as embryonic development, behaviour, gene order and gene expression; higher-level relationships remained stable when only morphological characters were included (DS-VI, which deactivated those characters). Although our results show increased congruence with molecular phylogenies for the deep divergences within Euarthropoda, they are less congruent with regards to some of the internal relationships of these clades, and in many cases resolve ‘traditional’ morphological groupings, such as a basal position for scorpions and opilionids within Arachnida ( Fig. 4g ) and the grouping of Entomostraca as a clade within the Pancrustacea ( Fig. 4h ). The arachnid example may reflect a paucity of fossils near the timing of cladogenesis. For example, many arachnid orders are well established in the Carboniferous and are assignable to extant clades; terrestrialization likely occurred in the late Cambrian–Ordovician [5] , but the fossil record before the Devonian is poor, and hence can contribute few informative character combinations to analyses. In the morphology-only data set (DS-VI), some extant internal nodes collapsed but the general relationships amongst larger clades, for example, Euchelicerata, remain consistent. Increased congruence with molecular results in our full data set analysis when compared with our extant-only analysis provides clear evidence that the addition of fossils improves the results of morphological parsimony analysis, as intermediate morphologies allow breaking up long branches and provide a root for character polarization. We hence advocate the inclusion of fossils in any large-scale phylogenetic analysis of morphological data. Taxon and character sampling The current data set is based on ref. 24 . The 173 taxa and 580 characters used therein ( Supplementary Note 1 ) were supplemented with a further 138 taxa and 173 characters ( Supplementary Note 2 ); the total data set consists of 311 taxa and 753 characters. Of these 311 taxa, two represent non-panarthropod ecdysozoans ( Caenorhabditis and Priapulus ) and were used as universal outgroups, and 25 represent non-arthropod Panarthropoda, including two extant tardigrades and two extant onychophorans. The remaining 284 arthropods included 194 fossils and 90 extant exemplars (the latter consisting of 3 pycnogonids, 21 euchelicerates, 13 myriapods, 13 hexapods and 40 crustaceans). Cladistic analysis All versions of this data set (see below) were converted into NEXUS file format [32] ( Supplementary Data 1 ) and analysed using TNT v.1.1. (Tree analysis using New Technology) [33] . The large size of the data set makes the probability of finding local optima very high and therefore necessitates the use of New Technology Search options [34] . These included 100 Random addition sequences with Parsimony Ratcheting [35] , Sectorial Searches, Tree Drifting and Tree Fusing [34] . Experimentation with these settings revealed that default options were sufficient for finding optimal trees. All characters were treated as non-additive (unordered) and weighted using both equal and implied character weighting options (see below). Nodal support was measured using Symmetric Resampling [36] . This measure is most appropriate to implied weights, because (unlike bootstrapping or jackknifing) it is not affected by character weighting and transformation costs [36] . Symmetric resampling used 1,000 replicates, each involving a New Technology search with a change probability of 33%. Nodal support values are expressed as Group present/Contradicted frequency differences ( Fig. 4 ). To determine the impact of both character and taxon inclusion, a set of experiments was undertaken in which either particular classes of characters (for example, characters associated with terrestrialization) or taxa were selectively deactivated (see main text). These subsets of the data were then rerun using the methodology outlined above. Given the large size of the data sets, it is computationally unfeasible to undertake selective higher-order taxon jackknifing. For this reason, individual taxa or selections of taxa were selected using a random number generator. Twenty-five random replicates were undertaken (DS-V). Implied weighting Justification for differential character weighting, particularly implied weighting, has been given elsewhere [20] , [24] , [37] . In summary, equal character weighting is only appropriate in analyses with no potential homoplasy, although this is rarely, if ever, the case. Most methods of differential character weighting require either a priori weighting or a posteriori weighting. Both of these require either an ad hoc assumption of character importance or reference to a current topology and thus can lead to circular reasoning, that is, weighting is based on a topology, which in turn was based on weighting. Implied weighting has been proposed as a method to overcome this logical impasse [37] . During implied weighing, characters are weighted during tree searches and the resultant Most Parsimonious Trees are compared to determine the maximum total character fit. The character fit is determined as a function of homoplasy such that those characters with most homoplasy will have a lower character fit. The most parsimonious tree is therefore the one with the greatest character fit. Unlike other character-weighting methods, which may produce a tree longer than those implied if characters were equally weighted, implied weighting is self-consistent, that is, it will only produce trees shorter under the weights they imply. Character fit can be adjusted using a concavity constant ( k ), where k determines how much a character is downweighted based on its level of homoplasy. The default option for TNT is k =3, a near-linear decreasing function, and is the constant preferred here, as it resolves relationships in favour of those with less homoplasy [34] , whereas a concavity constant <3 would resolve relationships in favour of more homoplasy, but increase the overall character usage. All analyses were undertaken using a variety of concavity constants (2, 3, 5 and 10) to determine the effect of character weighting on hypotheses of relationship. How to cite this article: Legg, D. A. et al . Arthropod fossil data increase congruence of morphological and molecular phylogenies. Nat. Commun. 4:2485 doi: 10.1038/ncomms3485 (2013).